Relationship of circulatingPlasmodium falciparumlifecycle stage to circulating parasitemia and total parasite biomass 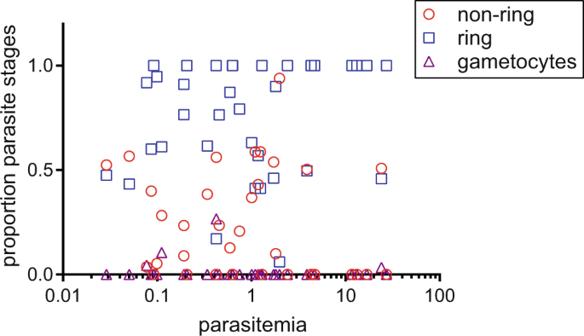Fig. 1: Circulating parasitemia does not correlate with circulating parasite age. Parasitemias for the 16 severe malaria samples and 19 uncomplicated malaria samples that were used for the differential gene expression analysis of the full transcriptome are plotted against the proportion of the circulating parasites estimated by our mixture model that were ring stages, asexual non-ring stages and gametocytes1. Source data are provided as a Source Data file. 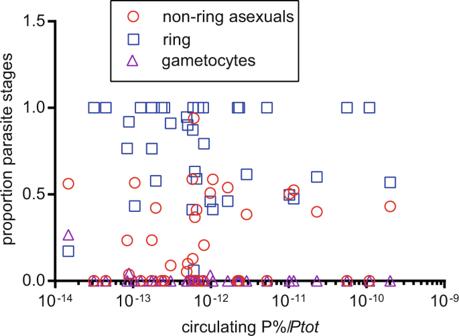Fig. 2: A relative measure of the proportion of total parasites that were circulating, i.e., the ratio of circulating parasitemia/calculated total parasite biomass (Ptot) does not correlate with proportions of circulating ring stage or asexual, non-ring stage parasites. Circulating parasitemia/Ptot from 37 malaria patient samples1plotted against the proportion of gametocytes, asexual non-ring stage parasites and ring stage parasites estimated by our mixture model from the parasite transcriptomes of each sample1. Source data are provided as a Source Data file. Further information on research design is available in the Nature Research Reporting Summary linked to this article.